Differential use of importin-α isoforms governs cell tropism and host adaptation of influenza virus Influenza A viruses are a threat to humans due to their ability to cross species barriers, as illustrated by the 2009 H1N1v pandemic and sporadic H5N1 transmissions. Interspecies transmission requires adaptation of the viral polymerase to importin-α, a cellular protein that mediates transport into the nucleus where transcription and replication of the viral genome takes place. In this study, we analysed replication, host specificity and pathogenicity of avian and mammalian influenza viruses, in importin-α-silenced cells and importin-α-knockout mice, to understand the role of individual importin-α isoforms in adaptation. For efficient virus replication, the polymerase subunit PB2 and the nucleoprotein (NP) of avian viruses required importin-α3, whereas PB2 and NP of mammalian viruses showed importin-α7 specificity. H1N1v replication depended on both, importin-α3 and -α7, suggesting ongoing adaptation of this virus. Thus, differences in importin-α specificity are determinants of host range underlining the importance of the nuclear envelope in interspecies transmission. Influenza virus replication involves interactions with cellular factors to which the virus has to adapt when transmitted to a new host. Thus, the haemagglutinin of avian viruses changes receptor specificity to allow entry into human cells [1] , [2] . Another cellular barrier is the nuclear envelope that needs to be overcome by influenza viruses. Adaptive mutations in the polymerase subunit PB2 and the nucleoprotein (NP) have been shown to enhance binding to importin-α, thereby promoting virus transcription and replication in the nucleus [3] . Importin-α is a constituent of the classical nuclear import pathway. It acts as an adaptor protein that recognizes the nuclear localization signal (NLS) of the cargo protein and is transported as a ternary complex with the importin-β receptor into the nucleus [4] . In humans and in chickens, six importin-α isoforms are known [5] , [6] , [7] , [8] , [9] . To determine whether the viral polymerase and NP discriminate between the different isoforms for nuclear import, we have analysed replication and pathogenicity of various avian and mammalian influenza viruses, including human H5N1 and recent H1N1v isolates, in importin-α-silenced cell cultures and importin-α-knockout mice. In this study, we show that avian influenza viruses undergo a switch in importin-α dependency upon avian–mammalian adaptation. For efficient virus replication, avian viruses depend on importin-α3, whereas mammalian viruses depend on importin-α7. These observations indicate that differences in importin-α specificity are determinants of host range highlighting the crucial role of the nuclear membrane in interspecies transmission. Differential importin-α specificities of influenza viruses Human and chicken importin-α isoforms vary in their amino-acid sequences from 82 to 99% identity; namely, α1 (82%), α3 (99%), α4 (98%), α5 (95%), α6 (94%) and α7 (94%) ( Supplementary Fig. S1 ). These data suggest that all importins show sufficient sequence divergence to potentially restrict interspecies transmission of influenza viruses. When individual importins were silenced in avian cells by small interfering RNA (siRNA; Supplementary Fig. S2a ), the highly pathogenic avian influenza virus (HPAIV) SC35 (H7N7) and its murine variant SC35M [10] grew to similar titres ( Supplementary Fig. S2b,c ) suggesting redundancy of chicken importins for influenza virus replication. In contrast, in importin-α-silenced human lung cells ( Fig. 1a ), SC35 growth was restricted by ≥1 log in importin-α1- and -α3-silenced cells ( Fig. 1b ). SC35M growth was not affected by importin-α3 silencing, but was strongly reduced (2 logs) in importin-α7-silenced human cells ( Fig. 1c ). Thus, in human cells, SC35 has a preference for importin-α3, whereas SC35M prefers importin-α7. Both viruses depend on importin-α1. The other importins appear to be redundant. 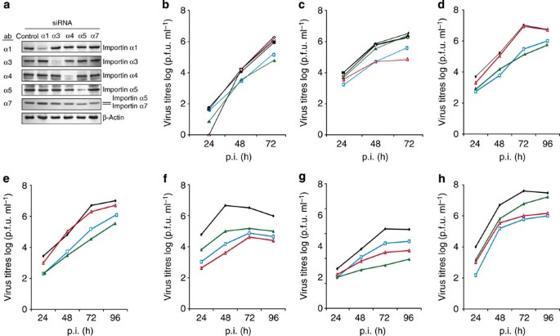Figure 1: Growth curves of avian and mammalian H7N7 mutant viruses in importin-silenced human cells. (a) Endogenous importins (α1–α7) were silenced using siRNA in human lung cells (A549). Importin-α7 antibody crossreacts with importin-α5. The doublet represents importin-α5 (upper band) and importin-α7 (lower band). (b–h) Virus growth in importin-α-silenced A549 cells infected with (b) SC35, (c) SC35M, (d) SC35-PB1SC35M, (e) SC35-PASC35M, (f) SC35-PB2SC35M, (g) SC35-NPSC35Mand (h) the mutant SC35-PB2701N-NP319K. Growth curves show controls (black, filled diamonds), α1 (blue, squares), α3 (green, filled triangles), α4 (black, filled squares), α5 (black diamonds) and α7 (red triangles) silenced cells. Figure 1: Growth curves of avian and mammalian H7N7 mutant viruses in importin-silenced human cells. ( a ) Endogenous importins (α1–α7) were silenced using siRNA in human lung cells (A549). Importin-α7 antibody crossreacts with importin-α5. The doublet represents importin-α5 (upper band) and importin-α7 (lower band). ( b – h ) Virus growth in importin-α-silenced A549 cells infected with ( b ) SC35, ( c ) SC35M, ( d ) SC35-PB1 SC35M , ( e ) SC35-PA SC35M , ( f ) SC35-PB2 SC35M , ( g ) SC35-NP SC35M and ( h ) the mutant SC35-PB2 701N -NP 319K . Growth curves show controls (black, filled diamonds), α1 (blue, squares), α3 (green, filled triangles), α4 (black, filled squares), α5 (black diamonds) and α7 (red triangles) silenced cells. Full size image To analyse the role of the polymerase and NP in the switch from importin-α3 to importin-α7 dependency upon avian–mammalian adaptation, we have assessed growth kinetics of SC35/SC35M single gene reassortants (SGRs) in importin-α-silenced cells. SC35M-PB1 (SC35-PB1 SC35M ) or -PA (SC35-PA SC35M ) had no effect on the acquisition of importin-α7 dependency ( Fig. 1d,e ). In contrast, SC35M-PB2 (SC35-PB2 SC35M ) and SC35M-NP (SC35-NP SC35M ) both gained importin-α7 dependency ( Fig. 1f,g ). All SGRs depend on importin-α3 ( Fig. 1d–g ). When we combined SC35M-PB2 and -NP mutations responsible for increased importin-α binding in general ( Supplementary Fig. S3 and ref. 3 ) in SC35-PB2 701N -NP 319K , dependency shifted from importin-α3 to importin-α7 ( Fig. 1h ). All reassortants depend on importin-α1 ( Fig. 1 ). Thus, the switch from importin-α3 to importin-α7 dependency is mediated by PB2-D701N and NP-N319K. Importin-α specificity has a regulatory role when several cargo proteins (viral and cellular) compete with each other for nuclear entry [11] . The distinct importin-α7 dependency of SGRs SC35-PB2 SC35M and SC35-NP SC35M ( Fig. 1f,g ), as well as the stronger interaction of PB2-D701N and NP-N319K with importin-α7 ( Supplementary Fig. S3 ), highlight the role of mammalian adapted PB2 and NP in the regulation of importin-α7 dependency. Pathogenicity and cell tropism in importin-α-knockout mice We next analysed virus infection in various importin-α-knockout mice, specifically those lacking α4, α5 and α7. Two different constructs were used for the importin-α7 gene knockouts, that is, animals lacked the entire importin-α7 gene (α 7 −/− ) or just the importin-β-binding domain (IBB) of importin-α7 essential for nuclear transport (α 7 Δ IBB/ Δ IBB ). After infection with SC35M (ref. 10 ), all wild-type (WT), importin-α4-deficient mice (α 4 −/− ) and importin-α5-deficient mice (α 5 −/− ) died ( Fig. 2a ). Interestingly, despite high infection doses, one-third of α 7 −/− and α 7 Δ IBB/ Δ IBB animals survived and started to regain weight 8 days post-infection (p.i.) ( Fig. 2a,b ). These findings show that the mouse-adapted virus depends specifically on importin-α7 to develop its full pathogenic potential. 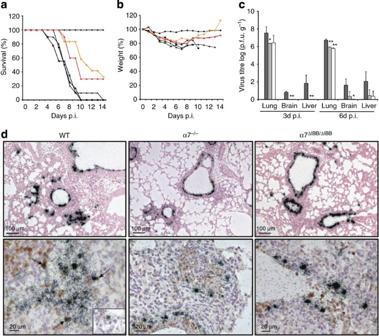Figure 2: Pathogenicity of SC35M in WT and importin-α-knockout animals. WT (black square;n=18), α4−/−(black triangle;n=16), α5−/−(black cross;n=16), α7−/−(red triangle;n=16) and α7ΔIBB/ΔIBB(orange circle;n=18) animals were infected with 100-fold LD50of SC35M. Control groups received PBS (black diamond). (a) Survival and (b) weight loss were monitored for 14 days. (c) Virus titres in the lung, brain and liver homogenates of controls (black columns) and infected WT (dark grey columns), α7−/−(light grey columns) and α7ΔIBB/ΔIBB(white columns) animals were determined by plaque assays. The error bars indicate the standard deviation of viral titres detected in three animals per time point. The detection limit was ≥30 p.f.u. (d)In situhybridization (upper panels) shows severe infection of epithelial cells with classical signs of primary viral pneumonia with extensive infiltration and destruction of the alveolae in WT mice (upper left panel) in contrast to mostly intact lung tissues of α7−/−or α7ΔIBB/ΔIBBanimals (upper middle and right panel). Double-labelling experiments (lower panels) demonstrate virus RNA-positive Mac-3+ macrophages in the lungs of WT mice (lower left panel, arrows and inset) but not in α7−/−or α7ΔIBB/ΔIBBanimals infected for 3 days (lower middle and right panel), respectively. The statistical significance of differences in lung titres of WT and importin-knockout animals were assessed by Student'st-test (*P<0.05; **P<0.01). Figure 2: Pathogenicity of SC35M in WT and importin-α-knockout animals. WT (black square; n =18), α4 −/− (black triangle; n =16), α 5 −/− (black cross; n =16), α 7 −/− (red triangle; n =16) and α 7 Δ IBB/ Δ IBB (orange circle; n =18) animals were infected with 100-fold LD 50 of SC35M. Control groups received PBS (black diamond). ( a ) Survival and ( b ) weight loss were monitored for 14 days. ( c ) Virus titres in the lung, brain and liver homogenates of controls (black columns) and infected WT (dark grey columns), α 7 −/− (light grey columns) and α 7 Δ IBB/ Δ IBB (white columns) animals were determined by plaque assays. The error bars indicate the standard deviation of viral titres detected in three animals per time point. The detection limit was ≥30 p.f.u. ( d ) In situ hybridization (upper panels) shows severe infection of epithelial cells with classical signs of primary viral pneumonia with extensive infiltration and destruction of the alveolae in WT mice (upper left panel) in contrast to mostly intact lung tissues of α 7 −/− or α 7 Δ IBB/ Δ IBB animals (upper middle and right panel). Double-labelling experiments (lower panels) demonstrate virus RNA-positive Mac-3+ macrophages in the lungs of WT mice (lower left panel, arrows and inset) but not in α 7 −/− or α 7 Δ IBB/ Δ IBB animals infected for 3 days (lower middle and right panel), respectively. The statistical significance of differences in lung titres of WT and importin-knockout animals were assessed by Student's t -test (* P <0.05; ** P <0.01). Full size image SC35M causes systemic infection including severe pneumonia and neurotropism in mice [12] . To study spread of infection and organ tropism in α 7 −/− and α 7 Δ IBB/ Δ IBB animals as compared with WT ( Fig. 2a,b ), we analysed virus titres in the lung, brain and liver. At day 3 p.i., high virus titres were detected in the lung, brain and liver of SC35M-infected WT mice ( Fig. 2c ). In contrast, in α 7 −/− and α 7 Δ IBB/ Δ IBB animals virus infection was restricted to the lung on day 3 p.i. ( Fig. 2c ). On day 6 p.i., high virus titres were detected in the lung, liver and brain of infected WT mice, whereas in α 7 −/− and α 7 Δ IBB/ Δ IBB mice infection was restricted mainly to the lung ( Fig. 2c ). It was previously reported that similar virus titres allowed systemic SC35M infection in mice that was mediated by spread through macrophages [12] . Interestingly, macrophages are infected in WT animals, whereas this was not the case in the lungs of α 7 −/− and α 7 Δ IBB/ Δ IBB mice ( Fig. 2d ). These data suggest that importin-α7 is important for virus spread to extrapulmonary organs, supporting the concept that importin-α specificity has a role in cell and organ tropism of influenza viruses. Importin-α3 to -α7-specificity switch upon mammalian adaptation We have extended our studies to other avian and mammalian influenza viruses of different subtypes. Virus growth of the HPAIV A/FPV/Rostock/1/34 (H7N1) was restricted in importin-α3-silenced cells ( Fig. 3a ), whereas the HPAIV A/Thai/KAN-1/04 (H5N1) isolated from a lethal human case [13] was not affected in importin-α3-silenced cells but reduced in importin-α7-silenced cells by 2 logs ( Fig. 3b ). Growth of the human A/Victoria/3/75 (H3N2) virus was also restricted in importin-α7-silenced cells ( Fig. 3c ). A/Sachsen-Anhalt/101/09 (H1N1v) and A/Hamburg/NY1580/09 (H1N1v) isolates from the 2009 pandemic were restricted in both importin-α3- and importin-α7-silenced cells ( Fig. 3d,e ). All viruses are dependent on importin-α1, whereas importin-α4 and -α5 appear to be redundant ( Fig. 3 ). These data support the concept that human adaptation of influenza viruses is also associated with the acquisition of importin-α7 specificity. 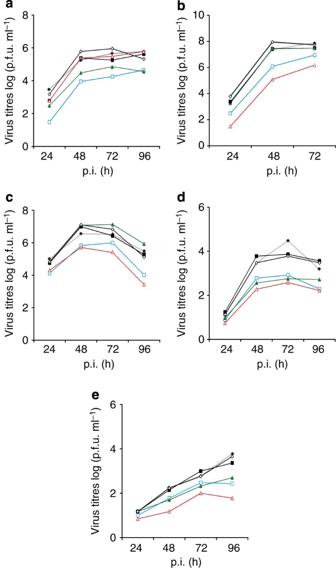Figure 3: Growth curves of various avian and human influenza viruses in importin-silenced human cells. Endogenous human importins (α1–α7) were silenced using siRNA in human lung cells (A549) and infected with (a) A/FPV/Rostock/1/34 (H7N7), (b) A/Thai/KAN-1/04 (H5N1), (c) A/Victoria/3/75 (H3N2), (d) A/Sachsen-Anhalt/101/09 (H1N1v) or (e) A/Hamburg/NY1580/09 (H1N1v). Growth curves show controls (black, filled diamonds), α1 (blue, squares), α3 (green, filled triangles), α4 (black, filled squares), α5 (black diamonds) and α7 (red triangles)-silenced cells. Figure 3: Growth curves of various avian and human influenza viruses in importin-silenced human cells. Endogenous human importins (α1–α7) were silenced using siRNA in human lung cells (A549) and infected with ( a ) A/FPV/Rostock/1/34 (H7N7), ( b ) A/Thai/KAN-1/04 (H5N1), ( c ) A/Victoria/3/75 (H3N2), ( d ) A/Sachsen-Anhalt/101/09 (H1N1v) or ( e ) A/Hamburg/NY1580/09 (H1N1v). Growth curves show controls (black, filled diamonds), α1 (blue, squares), α3 (green, filled triangles), α4 (black, filled squares), α5 (black diamonds) and α7 (red triangles)-silenced cells. Full size image H1N1v and H5N1 pathogenesis in importin-α7-knockout mice We next assessed the pathogenicity and cell tropism of the H5N1 and the H1N1v isolates in importin-α7-knockout mice. All WT animals infected with the H5N1 virus showed systemic virus spread with high titres in lung, liver and blood, and died on day 9 p.i. ( Fig. 4a,b ; Supplementary Fig. S4a ). All H5N1-infected α 7 −/− mice died, too, but virus titres were reduced in the liver and gut and abolished in blood ( Fig. 4a,b ). No significant differences were observed in the weight loss of α 7 −/− and WT mice ( Supplementary Fig. S4a ). H1N1v was shown to be pathogenic for several mammalian species [14] , [15] , [16] . Accordingly, WT mice infected with A/Sachsen-Anhalt/101/09 (H1N1v) showed lethal pneumonia with high virus titres only in lungs ( Fig. 4c,d ; Supplementary Fig. S5b ). Infection with A/Hamburg/NY1580/09 (H1N1v) was also lethal ( Fig. 4e ), but revealed systemic spread with high virus titres in the lung, liver, brain and gut ( Fig. 4f ; Supplementary Fig. S5c ). The genetic determinants responsible for the differences in the spread of infection in different strains of H1N1v-infected WT animals ( Fig. 4d,f ) remain to be investigated. However, in α 7 −/− and α 7 Δ IBB/ Δ IBB mice virus loads were reduced and confined to the lung ( Fig. 4d,f ; Supplementary Fig. S5 ), and all animals survived infection with marginal weight loss ( Fig. 4c,e; Supplementary Fig. S4b,c ). Interestingly, in H5N1- and H1N1v-infected importin-α7-knockout mice only single macrophages were found to be infected compared with WT animals, in which infected macrophages were abundant ( Supplementary Fig. S5 ). Taken together, these results support the view that the high pathogenicity and cell tropism of H1N1v and H5N1 isolates in mice depends on importin-α7 expression. 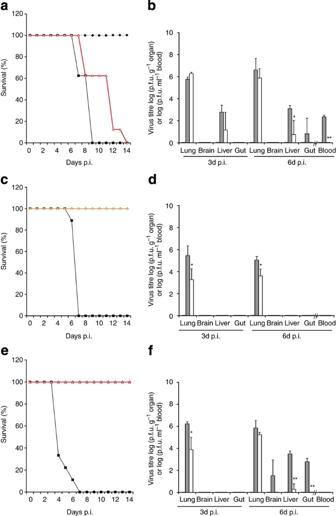Figure 4: Pathogenicity of H5N1 and H1N1v viruses in WT and importin-α7-knockout animals. WT (black square;n=16), α7−/−(red triangle;n=16) or α7ΔIBB/ΔIBB(orange triangle;n=16) animals were infected with 50-fold LD50of (a,b) A/Thai/KAN-1/04 (H5N1), (c,d) 10-fold LD50of A/Sachsen-Anhalt/101/09 (H1N1v) or (e,f) 100-fold LD50of A/Hamburg/NY1580/09 (H1N1v). Control groups received PBS (black diamond). (a,c,e) Survival was monitored for 14 days. (b,d,f) Virus titres in the lung, brain and liver homogenates and in the blood of infected WT, α7−/−and α7ΔIBB/ΔIBBanimals were determined by plaque assays. The statistical significance of differences in lung titres of WT and importin-knockout animals were assessed by Student'st-test (*P<0.05; **P<0.01). The error bars indicate the standard deviation of viral titres detected in three animals per time point. The detection limit was ≥30 p.f.u. Figure 4: Pathogenicity of H5N1 and H1N1v viruses in WT and importin-α7-knockout animals. WT (black square; n =16), α 7 −/− (red triangle; n =16) or α 7 Δ IBB/ Δ IBB (orange triangle; n =16) animals were infected with 50-fold LD 50 of ( a , b ) A/Thai/KAN-1/04 (H5N1), ( c , d ) 10-fold LD 50 of A/Sachsen-Anhalt/101/09 (H1N1v) or ( e , f ) 100-fold LD 50 of A/Hamburg/NY1580/09 (H1N1v). Control groups received PBS (black diamond). ( a , c , e ) Survival was monitored for 14 days. ( b , d , f ) Virus titres in the lung, brain and liver homogenates and in the blood of infected WT, α 7 −/− and α 7 Δ IBB/ Δ IBB animals were determined by plaque assays. The statistical significance of differences in lung titres of WT and importin-knockout animals were assessed by Student's t -test (* P <0.05; ** P <0.01). The error bars indicate the standard deviation of viral titres detected in three animals per time point. The detection limit was ≥30 p.f.u. Full size image Influenza viruses need to cross species barriers to adapt to new hosts. The first barrier to be overcome is the cell membrane. Therefore, the haemagglutinin of avian influenza viruses changes receptor specificity to allow entry into human cells [1] , [2] . In this study, we show that the nuclear membrane is a second major barrier that influenza viruses need to overcome upon adaptation to the mammalian host. Differences in importin-α specificities are determinants of host range underlining the crucial role of the nuclear membrane in interspecies transmission. The nuclear barrier is overcome by avian influenza viruses by gaining adaptive mutations in PB2 and NP, leading to a switch from importin-α3 to importin-α7 specificity upon mammalian adaptation. Importin-α specificity becomes important when several viral and cellular cargo proteins compete with each other for nuclear entry [11] . It has been previously reported that PB2 of A/Thai/KAN-1/04 (H5N1) binds poorly to human importin-α7, whereas PB2 of A/Victoria/3/75 (H3N2) shows strong binding to human importin-α5 (ref. 17 ). Consistent with the findings described here and by others [11] , [18] , PB2 binding to and PB2 specificity for a given importin-α isoform do not necessarily correlate, because binding to importin-α isoforms is primarily mediated by the NLS but specificity is dependent on both the NLS and protein context. H1N1v viruses have retained the avian signature at PB2 positions 627 (ref. 19 ) and 701 (ref. 10 ), with compensating adaptive mutations at positions 590 and 591 ( Supplementary Fig. S6a ) [20] . Our observation, that H1N1v viruses show specificity for both, importin-α3 and -α7, is therefore of particular interest, as it suggests ongoing adaptation. The role of particular amino acids of PB2 and NP ( Supplementary Fig. S6 ) in determining dependency on importin-α3 and -α7 needs to be further investigated. The specificity of avian viruses for importin-α3 is of particular interest in the light of the high identity (99%; Supplementary Fig. S1 ) of this importin in avian and mammalian cells ( Supplementary Fig. S7 ). Thus, it seems that interaction with importin-α3 facilitates the initial stage of interspecies transmission of the avian virus and paves the way for adaptation to the mammalian host. Importin adaptation of the polymerase promotes not only interspecies transmission but also enhances pathogenicity. The H5N1 isolate analysed here contains the adaptive mutation PB2-701N supporting the view that it is at least partially adapted to humans. However, even with significantly reduced overall virus titres, yet 100% lethality, the effect of importin-α7-knockout on H5N1 pathogenicity was only marginal ( Fig. 4a,b ; Supplementary Fig. S5 ). These observations indicate that reducing virus load in α 7 −/− animals is not sufficient to reduce H5N1 lethality and that other factors, such as aberrant immune responses [21] , are also involved and need to be considered in H5N1 therapy. Our findings highlight the requirement of the nuclear transport machinery component importin-α7 in influenza host adaptation. However, these findings do not exclude the possibility that importins might have additional functions after nuclear entry such as directly affecting virus replication itself, as suggested before [17] . Clearly, further investigation is needed to understand the selective pressure in humans for influenza viruses to adapt to importin-α7. Numerous cellular proteins are known to interfere with virus replication, and knockout of these genes increases host susceptibility to infection [22] , [23] , [24] , [25] , [26] , [27] . In contrast, here we found that susceptibility of an animal can be reduced if a host factor is switched off. Importin-α7-knockout mice are phenotypically indistinguishable from WT animals. Mitigation of influenza virus infection by transient downregulation of importin-α7 may therefore be a strategy with therapeutic potential. Cells and viruses A549 (human lung carcinoma) and DF1 (chicken fibroblasts) cells were grown in DMEM (Dulbecco's minimal essential medium) supplemented with 10% FCS (fetal calf serum; Gibco). The recombinant viruses SC35, SC35M, the SGRs thereof SC35-PB1 SC35M , SC35-PA SC35M , SC35-PB2 SC35M and SC35-NP SC35M , and the mutant SC35-PB2 701N -NP 319K were propagated in embryonated chicken eggs, as described before [10] . Avian A/FPV/Rostock/1/34 (H7N1) was propagated in embryonated chicken eggs. Human isolates A/Victoria/3/75 (H3N2), 2009 pandemic A/Sachsen-Anhalt/101/09 (H1N1v) and A/Hamburg/NY1580/09 (H1N1v), as well as the human H5N1 isolate A/Thai/KAN-1/04 (H5N1) [28] , were grown on MDCK (Madin-Darby canine kidney) cells. A/Sachsen-Anhalt/101/09 (H1N1v) was kindly provided by Brunhilde Schweiger (Robert-Koch-Institut, Berlin). All H1N1v isolates were tested for the absence of other viruses, such as herpes viruses (herpes simplex virus type 1 and 2, varizella-zoster virus, cytomegalovirus and Epstein–Barr virus), enterovirus, influenza B virus and human parechovirus by PCR to exclude unwanted contamination. siRNA sequences and siRNA transfection siRNA corresponding to human and chicken importin-α1, -α3, -α4, -α5 and -α7 were designed using the siDesign Center from Dharmacon Research and were obtained from Sigma Proligo. The siRNA sequences targeting the human and chicken importins are shown in Supplementary Table S1 . For transfection, we seeded cells in 24-well plates to 60–70% confluency and used 3 μg siRNA mixed with Lipofectamine 2000 (Invitrogen) according to the manufacturer's protocols. The medium was replaced with fresh growth medium at 4–6 h post-transfection and cells were incubated for a further 48 h. Cells were lysed 48 h after siRNA transfection with lysis buffer (50 mM Hepes, pH 8.0, 25% glycerol, 0.5% NP-40, 200 mM NaCl, 0.07% β-mercaptoethanol, 1 mM phenylmethylsulphonyl fluoride, 1 tablet protease inhibitor cocktail (Roche) in a volume of 10 ml) and lysates were subjected to SDS–PAGE followed by Western blot analysis. Membranes were incubated with previously described antibodies against importins α1–4 (Abcam), α5 (Invitrogen) and α7 (ref. 11 ). As an internal standard, β-actin was determined with specific antibodies (Abcam). Proteins were detected by chemiluminescence (Amersham). The results shown are representatives of three independent experiments. Growth curves DF1 or A549 cells were transfected with siRNA as described above and infected 48 h after siRNA transfection with virus at a multiplicity of infection of 0.001 for multi-cycle replication. At time points 0, 24, 48, 72 and 96 h p.i., supernatants were collected and plaque titres determined on MDCK cells. The detection limit of the plaque titration was ≥30 p.f.u. The growth curves shown are the average result of four to six independent experiments. Immunoprecipitation assays 293T cells were co-transfected with 5 μg of pHW2000-SC35-PB2, SC35-PB2-D710N, SC35-NP or SC35-NP-N319K, as well as with 2 μg of Flag-tagged human pcDNA-importin-α1, -α3 or -α7. After 48 h of transfection, cells were lysed as described before [3] . Immunoprecipitation was performed using EZ view Red ANTI-FLAG M2 affinity gels (Sigma) and eluted using a FLAG peptide (Sigma) according to the manufacturer's protocol. Importins were stained with a Flag-antibody, and PB2 staining was performed with monoclonal antibodies, kindly provided by Juan Ortin [29] . NP staining was performed as described before [3] . Flag-tagged human importin constructs were kindly provided by Peter Palese [30] . Generation of importin-α-knockout mice A detailed description of the generation of these mice will be described elsewhere (R.F. et al ., unpublished data). Generation of importin- α5 −/− mice was described previously [31] . Animal experiments The animal experiments were performed according to the guidelines of the German animal protection law. All animal protocols were approved by the relevant German authority, the Regierungspräsidium Gießen and the Behörde für Stadtentwicklung und Umwelt Hamburg. WT (littermates from the corresponding breeding) and importin-α-knockout animals were anaesthetized with ketamine-xylazine (100 and 10 mg kg −1 , respectively) and inoculated intranasally with 50 μl of virus diluted in PBS. Animals were infected using 100-fold lethal dose 50 (LD 50 ) of SC35M (MLD 50 =log 2.8 p.f.u. ml −1 ) [10] , 50-fold LD 50 of A/Thai/KAN-1/04 (H5N1) (MLD 50 =log 0.33 p.f.u. ml −1 ), 10-fold LD 50 of A/Sachsen-Anhalt/101/09 (H1N1v) (MLD 50 =log 4.25 p.f.u. ml −1 ) or 100-fold LD 50 of A/Hamburg/NY1580/09 (H1N1v) (MLD 50 =log 3.5 p.f.u. ml −1 ), respectively. For detection of virus titres in infected organs and histopathology, three mice per group for each time point were killed at days 3 and 6 p.i. Virus titres were determined in homogenates of the lung, brain and liver tissues by plaque assays. Blood was taken by submandibular punctuation at days 3 and 6 p.i. The remaining animals were observed for 14 days after infection for weight loss and survival. In situ hybridization Influenza viral RNA in tissues was detected using single-stranded 35 S-labelled viral RNA probes, which were synthesized from a pBluescript II KS+ vector containing a fragment of the NP gene (nt 1,077–1,442) of A/FPV/Rostock/34 (H7N1) [32] or the corresponding fragment from A/Hamburg/NY1580/09 (H1N1v). Linearization of this plasmid with Hin dIII or Kpn I, respectively, and subsequent T7 RNA polymerase transcription produced an antisense RNA probe suited to detect NP-specific viral RNA. Control RNA probes were obtained from the vector containing the dual-promoter plasmid of coxsackievirus B3 (pCVB3-R1) [33] . Pretreatment, hybridization and washing conditions of dewaxed 5-μm paraffin tissue sections were performed as described previously [33] . Slide preparations were subjected to autoradiography, exposed for 3 weeks at 4 °C and counterstained with haematoxylin and eosin. Concurrent immunohistochemistry and in situ hybridization To investigate whether macrophages contain influenza genomes, tissue sections were processed by immunohistochemistry using a rat anti-mouse antibody recognizing Mac-3 (Becton Dickinson), which was followed by in situ hybridization for the detection of influenza viral RNA sequences (see previous section) as described previously [34] . Phylogenetic analysis From the GenBank we downloaded the protein sequences of human and chicken importin-α1, -α3, -α4, -α5, -α6 and -α7 (accession numbers for human importin-α1, -α3, -α4, -α5, -α6 and -α7: NM_002266, NM_002268, NM_002267, NM_002264, NM_002269, NM_012316; accession numbers for chicken importin-α1, -α3, -α4, -α5, -α6 and -α7: XM_415672, XM_422815, XM_417065, XM_416496, XM_419770, XM_417803) and aligned them using the Clustal X program (EMBL-EBI). The sequence of XM_417065 was corrected by sequencing newly isolated complementary DNA (cDNA) clones of chicken importin-α4 (see below). For tree calculation, we used the Clustal X and TreeView (EMBL-EBI) programs. Cloning of chicken importin-α4 Chicken importin-α4 (KPNA3) cDNA was cloned from RNA isolated from chicken UMNSAH/DF-1 cells and is available in GenBank (accession GQ228553) as a partial coding sequence. The protein, importin-α4 (ACS92710.1), is 498 amino acids long. It is uncertain whether this sequence includes the initiator methionine at residue 2 as N-terminal amino-acid sequence information is unavailable and 5′ RACE was not performed. This sequence corrects a predicted importin-α4 mRNA sequence (accession XM_417065.2) derived from chicken genomic DNA. Sequencing of H1N1v The PB2 and NP gene segment of the A/Hamburg/NY1580/09 (H1N1v) strain was sequenced as described before [35] and deposited in GenBank under the accession nos. GU480807 and HM598305. How to cite this article: Gabriel, G. et al . Differential use of importin-α isoforms governs cell tropism and host adaptation of influenza virus. Nat. Commun. 2:156 doi: 10.1038/ncomms1158 (2011).